A single evolutionary innovation drives the deep evolution of symbiotic N2-fixation in angiosperms Symbiotic associations occur in every habitat on earth, but we know very little about their evolutionary histories. Current models of trait evolution cannot adequately reconstruct the deep history of symbiotic innovation, because they assume homogenous evolutionary processes across millions of years. Here we use a recently developed, heterogeneous and quantitative phylogenetic framework to study the origin of the symbiosis between angiosperms and nitrogen-fixing (N 2 ) bacterial symbionts housed in nodules. We compile the largest database of global nodulating plant species and reconstruct the symbiosis’ evolution. We identify a single, cryptic evolutionary innovation driving symbiotic N 2 -fixation evolution, followed by multiple gains and losses of the symbiosis, and the subsequent emergence of ‘stable fixers’ (clades extremely unlikely to lose the symbiosis). Originating over 100 MYA, this innovation suggests deep homology in symbiotic N 2 -fixation. Identifying cryptic innovations on the tree of life is key to understanding the evolution of complex traits, including symbiotic partnerships. Symbiotic associations are among the most decisive drivers of ecological diversification, occurring in every aquatic and terrestrial habitat on earth [1] , [2] . Molecular tools have allowed us to identify remarkable radiations of symbiotic partnerships across diverse ecological conditions [3] , [4] , but it is unknown whether the regulatory mechanisms underlying such partnerships evolved repeatedly or are based on pre-existing ancestral pathways [5] . In general, traits arising from symbiotic partnerships require complex coordination between different species [6] , [7] and are typically characterized by a diversity of types and symbiotic states. This type of complex coordination is especially evident in the symbiosis between angiosperms and their N 2 -fixing bacterial symbionts that has evolved in thousands of plant species [8] , [9] . Although progress has been made in cataloguing the distinct morphologies and diverse microbial partnerships characterizing N 2 -fixing symbioses [6] , [10] , [11] and in the molecular mechanisms regulating the symbiosis in some plant species [12] , [13] , [14] , [15] , it is unknown how all this novelty was generated. Such diversity and wide taxonomic distribution could suggest multiple, independent regulatory circuits that arose de novo . Alternatively, there may be a shared mechanism underlying the evolution of these interactions. The latter view is consistent with the ‘predisposition’ hypothesis, which asserts that about 100 million years ago (MYA) certain angiosperms (the so-called N 2 -fixing clade) evolved a predisposition towards the evolution of nodulation [8] , [9] . Such a shared mechanism is conceptually analogous to the deep homology among complex animal organs, for example, eyes or limbs that are based on highly conserved, underlying regulatory circuits [5] . The concept of deep homology in the evolution of symbiotic N 2 -fixation has important implications for the conservation of regulatory mechanisms and also for the ongoing attempts to transfer the capacity for nodulation to non-fixing crops, such as rice, wheat and maize [16] , [17] . If there is no deep symbiotic homology, there are potentially multiple pathways towards achieving nodulation. However, if the phylogenetic history of the symbiosis does contain evidence of a deep homology, this predicts the existence of a single shared symbiotic trait among extant N 2 -fixing angiosperms. A deeply conserved ‘symbiotic N 2 -fixation’ pathway could then be identified using a cross-species comparative framework [18] , [19] . Qualitative reconstructions of the deep evolution of symbiotic N 2 -fixation in early angiosperms [8] , [9] as well as detailed phylogenetic analyses of symbiotic N 2 -fixation evolution at lower taxonomic levels [20] , [21] , [22] , [23] have greatly increased our understanding of N 2 -fixation history and have helped to generate evolutionary scenarios similar to that of the N 2 -fixation predisposition hypothesis [8] , [9] . However, until now quantitative phylogenetic reconstruction of the deep evolutionary history of the N 2 -fixing symbiosis has been difficult because of three main constraints. First, researchers were lacking a global angiosperm phylogeny with a comprehensive coverage of angiosperm diversity at the species level. Such species level detail is crucial because of the high number of losses and gains of the symbiosis within N 2 -fixation families [9] , [24] . This had prevented scientists from accurately mapping nodulation across extant plant species. Second, researchers have lacked a single, comprehensive database of global plant species capable of hosting N 2 -fixing symbionts. Lastly, current models of trait evolution have largely assumed homogenous processes to occur across an entire phylogeny and have thus been unable to account for variation in evolutionary rates [25] . This means that until recently, we have not been able to accurately detect subtle changes in rates of evolution or in ancestral symbiotic states over large phylogenies containing thousands of species. As a result, we have not yet been able to provide an explicit and quantitative reconstruction of the major events driving the origin of symbiotic N 2 -fixation. We resolve these three constraints by compiling the largest database of N 2 -fixing angiosperms and then mapping this data set onto the most up-to-date phylogeny of global angiosperms (32,223 species) [26] . We use a recent phylogenetic approach that permits among-lineage variation in the speed of character evolution [25] to infer rates of evolution and reconstruct ancestral states. Our aim is to map the evolution of symbiotic N 2 -fixation over the deep evolutionary history (over 200 MYA) of global angiosperms and ask whether a single evolutionary event or multiple pathways lead towards the evolution of nodulation in flowering plants. We find evidence of deep homology in the evolution of symbiotic N 2 -fixation. We pinpoint on the phylogeny the emergence of a single, cryptic precursor shared by all extant angiosperms capable of hosting N 2 -fixing symbionts, quantitatively confirming the N 2 -fixation predisposition hypothesis [8] . We then reconstruct the evolutionary history of this symbiotic precursor and map its current distribution across extant angiosperms. Our comprehensive reconstruction allows us to (i) identify non-fixing plant species alive today that are likely to still retain the precursor, and thus represent interesting model systems for introducing N 2 -fixation symbioses into crops and (ii) analyse the subsequent evolution of a symbiotic state we call ‘stable fixers’ (clades in which plants are extremely unlikely to lose symbiotic N 2 -fixation). More generally, we suggest that large-scale quantitative phylogenetic reconstruction methods will emerge as a crucial tool to study the evolution of symbioses and complex traits. N 2 -fixation data, plant phylogeny and trait reconstruction After compiling a comprehensive N 2 -fixation database of 9,156 angiosperm species, we identified 3,467 species that overlapped with the global angiosperms phylogeny [26] . Using these species, we tested the simplest model of symbiosis evolution, which assumes (i) direct evolution in angiosperms of N 2 fixing and direct loss [27] , and (ii) homogenous evolutionary processes across all branches analysed. This binary model was compared with a series of five ‘Hidden-Rate’ models [25] of increasing complexity that allowed for (i) heterogeneity in the speed of evolution and (ii) the possibility of intermediate steps before the origin of the trait itself. We used AICc (corrected Akaike Information Criterion) to determine which model best describes the character state distribution data. We did not assume any model structure a priori , but let the data drive model selection. 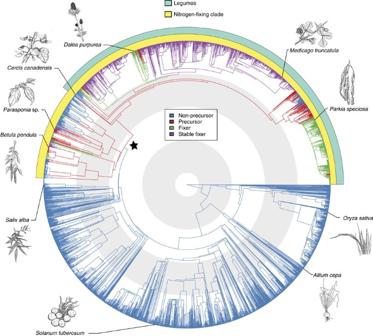Figure 1: Angiosperm phylogeny of 3,467 species showing reconstruction of node states. Branches are coloured according to the most probable state of their ancestral nodes. A star indicates precursor origin. Turquoise and yellow band indicate the legumes and the so-called nitrogen-fixing clade, which contains all known nodulating angiosperms8,9. Grey and white concentric circles indicate periods of 50 million years from the present. The positions of some important angiosperms are indicated with drawings (illustrations by Floortje Bouwkamp). Evolution of N 2 fixing is preceded by a necessary precursor The model that best explained the distribution of N 2 -fixation (AICc weight 55.5%) was a heterogeneous rate model with a single and necessary intermediate state in the path towards nodulation ( Supplementary Table 1 , Supplementary Fig. 1 ). In modelling terms, this means a plant species needs to move to a different rate class before it can evolve an N 2 -fixing character state (Methods). In biological terms, this intermediate state represents a precursor, an evolutionary innovation that must precede the evolution of a specific trait [28] , [29] , [30] , [31] . Our model identified several other important characteristics of N 2 -fixation ancestral states. First, a species that is in the precursor state is roughly 100 times more likely to evolve a functioning N 2 -fixation state (0.91 transitions per 100 million lineage years) than a non-precursor is to evolve a precursor (0.01 transitions per 100 million lineage years). Second, the precursor state is relatively easily lost, as evidenced by a high rate of disappearance of this state (1.25 transitions per 100 million lineage years). Third, our model identified a symbiotic state we call ‘stable fixer’ in which once acquired, an angiosperm lineage is extremely unlikely to lose the capacity for symbiotic N 2 -fixation (0.02 transitions per 100 million lineage years versus 1.17 for regular N 2 fixers). The symbiotic N 2 -fixation precursor evolved only once We mapped the likelihoods of being in each of the four symbiotic states (non-precursor, precursor, fixing and stable fixer) onto a time-scaled phylogenetic tree to identify the most important transitions in symbiotic N 2 -fixation evolution ( Fig. 1 , Supplementary Data 1 for expanded version including species names). Our model unambiguously pinpoints the single origin of the precursor within the Fabidae (also known as Rosids I) slightly over 100 MYA and at the base of the four orders comprising the N 2 -fixing clade (Fabales, Rosales, Cucurbitales and Fagales) [8] , [9] , [32] , subsequently leading to multiple emergences of nodulation capacity. We calculated the expected numbers of the major state transitions over our full phylogeny and confirmed the precursor state evolved only once ( Table 1 ) in the ~200 million year angiosperm history. Figure 1: Angiosperm phylogeny of 3,467 species showing reconstruction of node states. Branches are coloured according to the most probable state of their ancestral nodes. A star indicates precursor origin. Turquoise and yellow band indicate the legumes and the so-called nitrogen-fixing clade, which contains all known nodulating angiosperms [8] , [9] . Grey and white concentric circles indicate periods of 50 million years from the present. The positions of some important angiosperms are indicated with drawings (illustrations by Floortje Bouwkamp). Full size image Table 1 Number of evolutionary events: origins and losses of precursor, fixing and stable fixing states. Full size table Symbiotic N 2 -fixation has multiple origins and losses Although there is one single precursor origin, we found ~8 subsequent origins of N 2 -fixation itself (8.15±2.47 s.d., over N =100 alternative angiosperm phylogenies, Table 1 ), leading to the evolution of distinct symbiosis types in the angiosperms (most notably those involving rhizobial bacteria and those with actinorhizal Frankia sp.). The dramatic differences in infection modes, nodule forms, symbiont identity and resource control processes among N 2 fixers [6] , [10] , [11] demonstrate that substantial diversification of nodulation types took place following the origin of the shared precursor. The N 2 -fixation state has also been lost ~10 times (9.93,±2.80 s.d., N =100), a frequency that is lower than that of precursor state loss, but which still indicates that nodulation capacity is vulnerable over evolutionary timescales. The precursor was retained for more than 100 million years Our quantitative ancestral state reconstructions allow us to trace the evolution of the precursor since its origin over 100 MYA. We found that once evolved, the precursor state is vulnerable to loss, with an estimated 16.71 separate losses (±3.21 s.d., N =100, Table 1 ), including various times within the legumes ( Fig. 1 ). This vulnerability suggests that the precursor itself does not confer a large fitness benefit; many lineages have lost the precursor and are unlikely to remain predisposed towards N 2 -fixation. However, despite this vulnerability, our reconstruction reveals that the precursor has been maintained in some angiosperm species for over 100 million years to the current day ( Fig. 1 ). For each of our analysed species, we then calculated the precise likelihood of still being in precursor state today ( Supplementary Data 2 ). 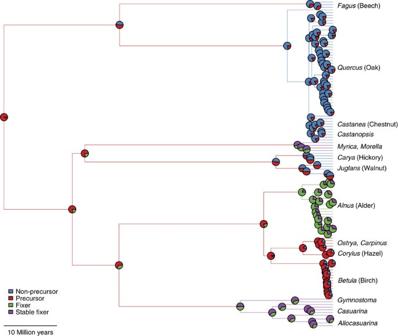Figure 2: Symbiotic states in the order Fagales. Pie charts indicate the likelihoods of a node being in each of four symbiotic states. Tree is labelled with genus names and associated common names. The Fagales clade highlights a range of potential transitions, including precursor loss (Fagus,Quercus, Castanea,Castanopsis), gain of fixing (Alnusetc) origins of stable fixing (Allocasuarina , Myricaand so on) as well as current precursor species (Corylus,Betulaand etc). We find that an extraordinarily diverse range of species across the angiosperm phylogeny are still highly likely to contain the precursor (for a selected subset see Table 2 ). This includes some unexpected non-legumes: for example, in the Fagales, all species of Betula , Corylus , Ostrya and Carpinus have high likelihoods of remaining in the precursor state ( Fig. 2 ). Table 2 Phylogenetically diverse subset of probable extant precursors and stable fixers. Full size table Figure 2: Symbiotic states in the order Fagales. Pie charts indicate the likelihoods of a node being in each of four symbiotic states. Tree is labelled with genus names and associated common names. The Fagales clade highlights a range of potential transitions, including precursor loss ( Fagus , Quercus, Castanea , Castanopsis ), gain of fixing ( Alnus etc) origins of stable fixing ( Allocasuarina , Myrica and so on) as well as current precursor species ( Corylus , Betula and etc). Full size image The precursor finding is robust to sources of uncertainty We confirmed that our main conclusion of a shared, single symbiotic N 2 -fixation precursor was robust to three sources of uncertainty. First, to verify that potential errors in our N 2 -fixation database would not affect our main conclusions, we re-ran our best model and the binary model ( Supplementary Table 1 ) while randomly discarding subsets of N 2 -fixation data. Even when we discarded up to 75% of the data points, our best model consistently performed better than the binary model ( Supplementary Fig. 2 ) and confirmed the emergence of a precursor in 98% of the model reruns. This is an important confirmation that our conclusions are not dependent on particular influential data points. Second, to address phylogenetic uncertainty in the underlying angiosperm phylogeny, we repeated our analyses over 100 alternative bootstrapped versions of the angiosperm phylogeny [26] , [33] and concluded that the evolutionary scenario including a necessary and single precursor was consistently recovered. We reached this conclusion because we found that for these 100 alternative phylogenies (i) the single precursor model consistently performed better than the binary model ( Supplementary Fig. 3 ), (ii) state transition rate estimates were highly similar ( Supplementary Fig. 4 ), (iii) a very similar mapping of ancestral states to the angiosperm phylogeny was obtained ( Supplementary Fig. 5 ) and (iv) similar numbers of evolutionary events were found ( Table 1 ). Lastly, we examined the second best reconstruction model (AICc weight of 42.9%, Supplementary Table 1 ) to test whether the precursor still emerged at the same point. Under this model, we confirmed there was also a necessary initial transition to a precursor state before evolution of symbiotic N 2 -fixation ( Supplementary Fig. 6 ) and phylogenetic mapping pinpointed this transition to the exact same origin ( Supplementary Fig. 7 ). These observations further strengthen our conclusion of a precursor being crucial to the evolution of symbiotic N 2 -fixation. Symbiotic N 2 -fixation is very stable in some clades Our quantitative phylogenetic framework identified a symbiotic state we call the stable fixers ( Supplementary Fig. 1 ). We catalogued 850 species that are more than 90% likely to be in this symbiotic state (see Table 2 for a subset of probable stable fixers). Our model suggests that this symbiotic fixing state has over 24 separate origins (24.53±4.79 s.d., N =100) and not a single expected loss (0.19±4.99 s.d., N =100), despite evolving over 50 MYA ( Fig. 1 , Table 1 ). In our second best model (see above), we also observe stable fixers (specifically in the Papilionoideae) , regular N 2 fixers and additionally a third category in which symbiotic N 2 -fixation is moderately stable (0.44 transitions per 100 million years compared with 0.02 for stable fixers and 1.79 for regular fixers under that model; Supplementary Fig. 6 ). Mapping of this second best model to our phylogeny reveals that the moderately stable fixing state, found for example in the Mimosoideae and in non-legume angiosperms associated with the actinorhizal N 2 -fixing symbionts, requires an intermediate precursor ( Supplementary Fig. 7 ). Our quantitative phylogenetic analysis demonstrates how symbiotic N 2 -fixation evolution was driven by a single and necessary evolutionary innovation. We show that in some clades this innovation was lost; in others, it laid the foundation for the emergence of a hugely successful class of nutrient symbioses that transformed the earth’s biogeochemistry [34] , [35] , [36] . These findings quantitatively confirm a shared predisposition underlying the evolution of all angiosperm symbiotic N 2 -fixation [8] . The single origin of this innovation implies a deep homology in symbiotic evolution, analogous to deep homology in complex organismal traits such as animal eyes and limbs [5] . The implication is that one basic regulatory circuit can produce a range of novel (co)evolutionary adaptations, not only to diverse ecological demands but also to divergent symbiotic partners. How do such complex traits evolve? Recent work on microbial genomes in an experimental evolution context has revealed three evolutionary stages of innovation: potentiation, actualization and refinement [37] , [38] . In the potentiating stage, one or multiple mutations arise, which enable the future evolution of the trait, but do not yet result in actual phenotypic changes. In our reconstruction, this step is analogous to the emergence of the N 2 -fixation precursor. Next, the actualizing mutation or mutations enable the emergence of the phenotype, often still in a rudimentary form. In our case, the multiple origins of N 2 -fixation states represent different actualizing mutations, producing various origins and diversity in N 2 -fixation types. Lastly, the stable fixers we identify in our model could represent multiple, probably distinct, refinement stages in which additional mutations are further fine-tuned and more efficiently expressed [37] , [38] . Linking these evolutionary stages to genetic changes in angiosperms over deep time is a major task. The identity of the N 2 -fixation precursor itself is among the greatest mysteries in the evolution of plant symbioses [8] , [9] and of mutualisms in general. Despite great progress in understanding the molecular details of the nodulation machinery [12] , [13] , [14] , [15] , [39] , [40] , an underlying precursor mechanism has yet to be confirmed. Unfortunately we lack the ‘frozen fossil records’ [41] used in microbiology that enable relatively easy identification of these types of mutations found in experimental evolution scenarios. It is well appreciated that the molecular machinery regulating interactions with N 2 -fixing bacteria greatly overlaps with the pathway mediating the more ancient fungal mycorrhizal symbiosis [6] , [42] , [43] . Given these similarities, the precursor may represent a modification to this pathway, with key shared steps mediating interactions with N 2 -fixing bacterial partners as well as fungi. For example, the well-characterized SymRK protein has been identified as a candidate [14] , [42] , but a non-N 2 -fixing clade version can likewise mediate symbiotic function [15] , suggesting it is unlikely to represent the precursor. Our analyses show that the precursor is very likely to be retained for over 100 MYA to the current day in some species ( Figs 1 and 2 , Table 2 and Supplementary Data 2 ). This suggests that any genetic modification represented by the precursor would not have had a major negative fitness impact. Rather, it is likely to have had some other fitness benefit before facilitating angiosperm nodulation, for example, modifications enabling discrimination of pathogenic bacteria from (free-living) N 2 fixers. In principle, the biological correlate of the cryptic precursor we have identified could be environmental in nature [25] , for example, facilitated by a shift in climate. However, an environmental factor would be shared by the many extant angiosperm lineages at the time of precursor evolution (~100 MYA) and would be expected to recur multiple times across the phylogeny, resulting in multiple independent precursor events. Instead, we identified only one singular event leading to the precursor state, despite a cumulative ~53 billion lineage years of evolution in our phylogeny. This lends support to the hypothesis that the transition represents a complex change in an underlying genetic or morphological trait specific to this lineage, but more evidence is needed. Quantitative phylogenetic reconstructions can substantially aid in the ongoing search for the N 2 -fixation precursor. Every plant species in our analysis has a likelihood of being in a particular symbiotic state (see Supplementary Data 2 ). This allows us to pinpoint previously unidentified precursor plant species alive today that are very likely to still retain the precursor. Candidate pathways in phylogenetically diverse species (see Table 2 ) can be catalogued and mapped onto the symbiotic N 2 -fixing phylogenetic tree ( Fig. 1 ) to test for overlap. The ancient single origin of the precursor means it is deeply homologous across the N 2 -fixing clade [5] , suggesting this highly conserved pathway could be identified using a cross-species comparative framework [18] , [19] . Overlapping symbiotic machinery (for example, signalling pathways, receptors) should be studied over as large a phylogenetically range of precursor species as possible ( Table 2 ). This should include various legume genera (for example, Nissolia , Parkia , Mora ), but also non-legumes such as those in the Cannabaceae (for example, Celtis , Trema ) and members of the Fagales ( Fig. 2 ). These distantly related species should share relatively few traits in addition to the true precursor, simplifying the search. In contrast, most current nodulation model species ( Medicago truncatula , Glycine max and Lotus japonicus ) have a high likelihood (>99%) of being stable fixers ( Supplementary Data 2 ). Although they can also contain the precursor, their relatively high taxonomic similarity gives a limited view of N 2 -fixation evolution and they are likely to share many traits in addition to the 100-MYA precursor, confusing the search. Species in the N 2 -fixing clade predicted to have lost the precursor should be included as negative controls in this comparative framework. A second key question arising from our analysis involves the underlying nature of the stable fixing symbiotic state. In biological terms, stable fixers are likely to be characterized by evolutionary innovations that have substantially increased symbiosis stability, not necessarily increased fixation rates. For example, the evolution of stable fixing in the Papilionoideae (~52 MYA) is predated by a whole-genome duplication ~58 MYA [44] . Whole-genome duplication potentially provided redundant copies of genes important in N 2 -fixation regulation, thereby reducing the risk of loss [45] , [46] . In contrast to the precursor, stable fixing species do not appear to share a single biological correlate. This is evidenced by ~24 origins of stable fixing under our best model ( Fig. 1 and Table 1 ). Under our second best model ( Supplementary Table 1 ), the stable fixer concept is more complicated, because two symbiotic states of stable fixing are predicted to have emerged ( Supplementary Fig. 6 ). One of these states matches the stable fixers as described in our best model ( Supplementary Fig. 1 ): this stable fixing state simply evolves from a regular fixing phenotype and is found mainly in the Papilionoideae . The additional (less stable) symbiotic state called a moderate fixer arising from our second best model, maps to both the Mimosoideae and actinorhizal fixers ( Supplementary Fig. 7 ) and requires a second, non-fixing precursor state before symbiotic N 2 -fixing phenotypes arise ( Supplementary Fig. 6 ). Under such an evolutionary scenario, this can be conceptualized as a second ‘potentiating’ mutation before ‘actualization’ in the moderate fixers. Studying potential genetic correlates of stable fixing for our best ( Supplementary Fig. 1 ) and second best ( Supplementary Fig. 6 ) model scenarios is important but challenging, because we do not expect there to be a single form of stable fixing. In contrast to the precursor, we anticipate multiple types of stable fixing, driven by multiple different mutations. Phylogenetic reconstruction allows us to pinpoint when the crucial modifications in the evolution of symbiotic N 2 -fixation occurred and to identify a range of symbiotic states, including current precursors and previously unidentified stable fixers. This type of reconstruction is beneficial for the long-standing goal of transferring N 2 -fixation into non-fixing crops, such as cereals [16] , [17] . We found, for example, that none of the major cereal grains are among the precursor species ( Fig. 1 and Supplementary Data 2 ), suggesting that modifying them for symbiosis with N 2 -fixing bacteria will be difficult until the specific precursor machinery is described. In contrast, a more obtainable goal may be to re-wire the symbiosis into species already primed with the precursor. Carpinus sp . (hornbeam) is an important timber crop with a 78.6–79.5% likelihood of retaining the precursor, whereas Parkia speciosa (bitterbean) is an important food crop in Asia and has a 85.0% likelihood of containing the precursor. More generally, the use of large-scale quantitative phylogenetic frameworks can help researchers identify deep homologies across divergent organisms, but also in relationships between organisms. We show that such frameworks [25] can help pinpoint the emergence of the major evolutionary stages of innovation (potentiation, actualization and refinement) [37] , [38] in the deep history of complex traits. Our work provides a clear example of the importance of cryptic putative precursors in the evolution of mutualistic partnerships and advocates for quantitative approaches to uncovering critical intermediate steps in (symbiotic) complex trait evolution. Compiling a comprehensive N 2 -fixation database To compile our database of current angiosperm symbiotic N 2 -fixation status, we used three main sources. First, we digitized data from the two most comprehensive volumes on legume nodulation [24] , [47] . Second, we obtained data from the TRY initiative that categorized plants based on confirmed N 2 -fixation status [48] . Our third data source was the Germplasm Resources Information Network (GRIN) database of the United States Department of Agriculture [49] . We supplemented these sources with data from the primary literature, focusing on taxa that were less represented in other databases. Plant species names were checked and inaccuracies resolved using the Taxonomic Name Resolution Service v3.1 (ref. 50 ) and, if necessary, manually verified using The Plant List [51] . The four data sources were then combined into a single database (9,156 species). In case of conflicts among data sources, we used the following preference order: primary literature>Legume volumes>TRY>GRIN. A total of 3,467 species overlapped with our angiosperm phylogeny and were analysed in detail. We pruned the full angiosperm phylogeny to these overlapping species for our analyses. We took care to manually evaluate as many potential errors in these data and in the plant species names as possible. Data for the species analysed for this paper can be found in the Supplementary Data 2 . This file contains all data used to construct models, the sources for these data, as well as the corrected state likelihoods for each species as inferred under the best model. The full data set of 9,156 species, including species not analysed in this study, has been archived at Dryad ( http://doi.org/10.5061/dryad.05k14 ). Full references to the various data sources can be found in Supplementary Table 2 . The angiosperm phylogeny To map the evolution of N 2 -fixation, we used a recently published phylogeny of 32,223 angiosperm species [26] , [33] . This phylogeny was generated using a maximum likelihood approach based on molecular data for seven loci (18S, 26S, ITS, matK, rbcL, atpB and trnLF); the tree building used the PHLAWD pipeline (ver. 3.3a) and total sequence alignment were performed using RAxML (ver. 7.4.1) [52] , [53] , [54] , [55] . The phylogeny was constrained based on several recent phylogenetic systematic treatments of seed plants [26] . Branch lengths were scaled based on a large fossil data set [26] . The full phylogeny can be found in Dryad [33] . Phylogenetic analysis of character state evolution To allow for variation in the speed of character evolution, we used an approach to infer rates of evolution and reconstruct ancestral states called ‘Hidden Rate Models’ (HRM) [25] . These models are a generalization of the covarion model of nucleotide substitution [56] , which allows for among-lineage heterogeneity in site-specific evolutionary rates of molecular sequence data. Classical methods of binary character state evolution (for example, the mk2-model [27] ) can be problematic at this phylogenetic scale, because they assume a single rate of evolution and loss of the focal trait. It is instead more realistic to assume that some angiosperm clades have a higher transition rate to and from symbiotic N 2 -fixation than other clades. HRMs allow for this heterogeneity in transition rates between the two character states (in this case N 2 fixing or non-fixing) of the focal trait over a phylogeny [25] . In HRMs, each node in the phylogeny has a character state, but is also in one of multiple rate classes (for example, Supplementary Fig. 1 ). Among rate classes, transition rates between the two character states can differ (that is, there is potential variation in the speed of evolution). A transition rate can be as low as zero, meaning the model can infer that a particular transition does not occur. At any point along the phylogeny, a species can either move to the other character state (horizontal transition in Supplementary Fig. 1 ) or it can move to another rate class (vertical transition in Supplementary Fig. 1 ). To accurately represent the evolution of a trait, it is necessary to infer transition rates for both of these potential transitions. These transition rates can be thought of as probabilities of moving or alternatively as a number of transition events per time unit (as represented in the main text). We used the R-package corHMM [25] to generate HRMs for our N 2 -fixing data set and the associated angiosperm phylogeny. For a given number of rate classes, this package infers transition rates between the various states in that HRM. It then reconstructs the most probable state of each node in the phylogeny, allowing us to map these states onto the phylogeny. Thus, for each node this framework provides the likelihoods of all of the potential states, summing up to 1. We used the marginal method to calculate states at each node [57] . To create our HRMs, we constrained the root node of the phylogeny to be a non-fixer (that is, the ancestral state of angiosperms). Relaxing this constraint does not result in different conclusions. Transition rates were not constrained in any way, meaning that they are free to be estimated at any value, including the zero bound. To sample the full multidimensional parameter space, we used 100 random restarts. We explored higher number of restarts, but this did not result in better model convergence; thus, for our main analyses 100 restarts were used. We generated HRMs assuming one to five rate classes, to allow for an exploration of a wide range of evolutionary scenarios. The HRM with only one rate class reduces to the basic mk2 model [27] and only assumes one gain and one loss rate. In addition, we generated a more limited case of the HRM framework, which requires a precursor state before the evolution of the focal character, but subsequently only allows one rate class for that character [28] . Whereas our other models do not assume a precursor (but allow for one), this limited case does assume the evolution of a precursor. To prevent model overfitting, we used AICc (AIC corrected for finite sample sizes) weights to determine which HRM best describes our character state distribution data ( Supplementary Table 1 ). For a family of models using the same character state database and phylogeny, AICc weights represent the conditional probability that a specific model provides the best explanation [58] . An HRM can infer a rate pattern in which a species must first make the transition to the next rate class, before making the transition from a non-fixing to a fixing character state. This pattern was observed under our best model ( Supplementary Fig. 1 ). The observed pattern is the modelling equivalent of a biological precursor: an innovation necessary for the evolution of the character but not the character phenotype itself. For this reason, we refer to the best HRM as the ‘single precursor’ model. Such a transition rate pattern is not inherent to HRMs: a direct transition from a non-fixing to a fixing character state (that is, not preceded by transition in rate class) is allowed under all models considered. For this reason, we have a posteriori assigned the states of our best model names that represent a biological interpretation (for example, ‘precursor’ and ‘stable fixer’). Number of evolutionary events The marginal ancestral reconstruction approach [57] constrains nodes to multinomial probabilities. As such, the expected number of major evolutionary events (gains and losses of precursors, fixing and stable fixing) over angiosperm phylogeny, can be estimated using the sum of the appropriate differences in state probability over the full phylogeny for each transition of interest. To exclude small fluctuations between two nodes that represent uncertainty in the underlying method rather than real evolutionary transitions, we used a cut-off value of 0.01 (that is, 1%) between two nodes. Under a maximum parsimony assumption, where on a given branch only one transition is possible between two nodes, this summation corresponds to the expected number of events that has occurred over the entire phylogeny given the estimated probabilities at each node ( Table 1 ). To obtain confidence estimates for these numbers, we repeated these steps for 100 bootstrap versions of our angiosperm phylogeny [26] , [33] , [59] , [60] and calculated s.d. and median values over the resulting distributions ( Table 1 ). These values indicate the extent to which the estimated event numbers are affected by phylogenetic uncertainty (see also below ‘Robustness to phylogenetic uncertainty’). Likelihoods of extant precursors and stable fixers To estimate the N 2 -fixing states of extant angiosperms, we used the character state likelihoods of the node directly ancestral to each species. Note that estimating extant states is only necessary for distinguishing non-fixing precursors from non-fixing non-precursor and for distinguishing stable fixers from fixers, as fixation can be directly observed in extant species. We then deducted the probability of a transition occurring on the terminal branch: the terminal branch length multiplied by the combined transition rates out of that state ( Supplementary Fig. 1 ). This correction is crucial because in some species the terminal branch may be tens of millions of years long. Consequently, without correction we would run the risk of strongly overestimating the likelihood an extant species still retains precursor or stable fixing state. Our more conservative approach is instead an underestimate of these likelihoods, because we only take into account the possibility of state loss over the terminal branch and not that of a gain of precursor or stable fixing state. Robustness to sampling uncertainty To account for uncertainty in the N 2 -fixation data set we compiled, we recalculated the basic binary and the single precursor models ( Supplementary Table 1 ) after dropping random species subsets from the full data set (retaining 25%, 33% or 50% of species). This helps account for false reports of nodulation or its absence found in the literature [61] . We repeated this procedure 100 times for each of these modified data sets and determined the difference in AICc between both models ( Supplementary Fig. 2 ). To test the null model that there is no pattern in the N 2 -fixation data, we furthermore generated 100 single precursor and 100 binary models using the same angiosperm phylogeny, but reshuffled the underlying N 2 -fixation data over all species ( Supplementary Fig. 2 ). This approach allows us to fix the proportions of fixers and non-fixers, but randomizes the actual distribution of nodulation over all species. Robustness to phylogenetic uncertainty A second source of uncertainty is in the phylogenetic relationships among the angiosperms. This includes, for example, various alternative estimates of phylogenetic relationships within the legumes, which are a subject of much current debate [62] . To test the robustness of our results with respect to this phylogenetic uncertainty, we used three alternative approaches using the 100 bootstrap phylogenies [26] , [33] , [59] , [60] containing a wide range of hypothesized evolutionary relationships in all clades, including within-legumes. First, we re-ran the single precursor and binary models for the 100 bootstrap phylogenies. We then determined the difference in AICc value for these re-runs ( Supplementary Fig. 3 ). Second, we analysed the transition rates between the four symbiotic states as they were calculated for each of these 100 phylogenies. We generated a histogram to show the distribution of these rates for each possible transition ( Supplementary Fig. 4 ). Third, we mapped the four symbiotic states as calculated using the median of the 100 alternative transition rates (rather than the transition rates inferred under the best phylogeny) to the angiosperm phylogeny ( Supplementary Fig. 5 ). Expanded phylogeny To allow the reader to find all individual species analysed in this study and identify interesting transition in the evolution symbiotic N 2 -fixation in more detail, we provide a supplementary expanded high-resolution phylogeny with individually readable species names at each branch tip ( Supplementary Data 1 ). This file is an expanded (>3 m × >3 m) version of Fig. 1 in the main text. In Supplementary Data 1 , branches are not only coloured according to the most probable state of the ancestral node, but also the exact state reconstruction per node is represented by a pie chart on each node. Colours represent the same states as in Fig. 1 . We also list N 2 -fixation status (as in our data set) between parentheses after each species name. How to cite this article: Werner, G. D. A. et al. A single evolutionary innovation drives the deep evolution of symbiotic N 2 -fixation in angiosperms. Nat. Commun. 5:4087 doi: 10.1038/ncomms5087 (2014).